APOBEC family mutational signatures are associated with poor prognosis translocations in multiple myeloma We have sequenced 463 presenting cases of myeloma entered into the UK Myeloma XI study using whole exome sequencing. Here we identify mutations induced as a consequence of misdirected AID in the partner oncogenes of IGH translocations, which are activating and associated with impaired clinical outcome. An APOBEC mutational signature is seen in 3.8% of cases and is linked to the translocation-mediated deregulation of MAF and MAFB , a known poor prognostic factor. Patients with this signature have an increased mutational load and a poor prognosis. Loss of MAF or MAFB expression results in decreased APOBEC3B and APOBEC4 expression, indicating a transcriptional control mechanism. Kataegis, a further mutational pattern associated with APOBEC deregulation, is seen at the sites of the MYC translocation. The APOBEC mutational signature seen in myeloma is, therefore, associated with poor prognosis primary and secondary translocations and the molecular mechanisms involved in generating them. Humans have evolved with the need to evade infection and as a consequence have developed DNA rearranging mechanisms to generate high affinity antibodies. An inevitable consequence of these processes is the generation of abnormal recombination events, leading to oncogene activation or tumour suppressor gene inactivation. Myeloma is a malignancy of plasma cells that develops later in life in which abnormal rearrangements at the Ig loci have been shown to be important initiating events. Consequently, studying the mechanisms underlying the development of translocations and their downstream effects can provide major insights into the aetiology of the disease [1] . Aberrant chromosomal translocations are seen in ∼ 40% of presenting patients and predominantly involve the IGH locus at 14q32 (ref. 2 ). There are five main partners to the IGH locus which are 4p, 6q, 11q, 16q and 20q all of which are considered as being classical myeloma translocations that are seen in close to 100% of the tumour population. These translocations result in the overexpression of an oncogene on the partner chromosome, which can be categorized using a translocation/cyclin classification [3] . The expression of the partner oncogene has a strong influence on the cell, resulting in changes to the genome and in a characteristic clinical behaviour of the disease. For example, the t(4;14) results in overexpression of FGFR3 and MMSET ( WHSC1 ) [4] . This translocation group is associated with a poor prognosis [5] , which is abrogated to some extent by the use of bortezomib treatment [6] . The overexpression of MMSET , which encodes a histone methyltransferase, results in gene-specific DNA hypermethylation, which is distinct from the other translocation groups [7] . The t(11;14) results in overexpression of CCND1 and the occurrence of this translocation is more likely in individuals carrying the G allele of the cyclin D1 SNP, rs9344, which affects its splicing pattern [8] . Both the t(4;14) and t(11;14) are relatively frequent events (12% and 15%, respectively) with the other three translocations occurring less frequently. The t(6;14) (1%) results in overexpression of CCND3 and the t(14;16) (4%) and t(14;20) (1%) result in overexpression of the transcription factors MAF and MAFB , respectively [3] . The ‘maf’ translocations are associated with a poor prognosis [9] . In initial sequencing studies of myeloma it has been noted that the spectrum of mutations fall into two groups, one of which is characterized by an APOBEC signature [10] . This signature comprises of C>T, C>G and C>A mutations in a TpC context and it has also been described in several cancers such as breast, pancreatic, chronic lymphocytic leukaemia (CLL) and B-cell lymphoma. This mutational signature comprises only a subset of samples, with the rest having a rather generic mutation signature with enrichment of C>T transitions at CpG dinucleotides, representing an intrinsic mutational process occurring as a result of the spontaneous deamination of methylated cytosine to thymine. Here we have performed whole exome sequencing on 463 patients with the addition of the Ig and MYC loci, to capture translocation breakpoints, copy number (CN) abnormalities and somatic mutations to determine how these affect mutation patterns in the plasma cell. We find that MYC translocations are indicative of poor prognosis and are associated with kataegis, translocation partner genes are mutated by AID in 15% of samples and mutation of CCND1 results in poor prognosis, and that APOBEC mutational signatures are associated with the t(14;16) and t(14;20) translocations and a high mutational load. Rearrangements at MYC are associated with a poor outcome Whole exome sequencing was performed on 463 presentation patients enroled into the Myeloma XI trial. 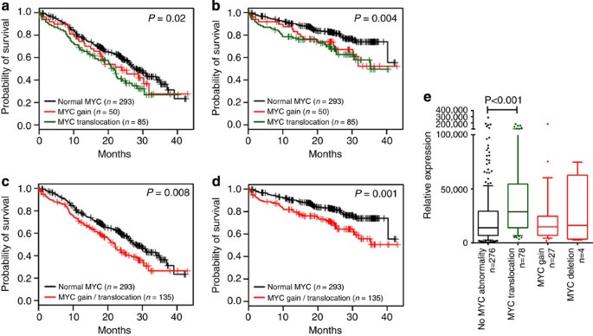Figure 1: MYC abnormalities affect survival. Progression free (a) and overall survival (b) of patients withMYCtranslocation, gain or no abnormality. Progression free (c) or overall survival (d) of patients comparing noMYCabnormality to those with either a translocation or gain of the locus. (e) relative expression ofMYCin samples with noMYCabnormality, a translocation at 8q24 or gain or loss of theMYClocus. The box and whisker plot shows the 10 and 90 percentiles (whiskers) and the median and 25 and 75 percentiles (box).Pvalues determined by log-rank test. Sequencing metrics are presented in Supplementary Table 1 . In addition to capturing the exome, extra baits were added covering the IGH , IGK , IGL and MYC loci to determine the breakpoints associated with translocations in these genes. These combined data allow us to examine the effect of translocations on the mutational spectra in myeloma. Using a combination of targeted capture and expression-based classification, we identified the five main translocation partners and those surrounding the MYC locus. Translocations were detected in 232 (50.1%) patients of which 59 patients (12.7%) had a t(4;14), 86 patients (18.6%) a t(11;14), 17 patients (3.7%) a t(14;16), 5 patients (1%) a t(6;14) and 4 patients (0.9%) a t(14;20). The remainder had translocations involving 8q24 with 21 (4.5%) patients having both a classical translocation and an 8q24 translocation and 62 (13.4%) having only an 8q24 translocation (of which 54 were hyperdiploid (HRD) and 8 were neither HRD nor had a classical translocation). Breakpoints are shown in Supplementary Fig. 1 and the distribution agrees with previously published results [11] . MYC translocations were found in 85 patients (18.4%). The most common partner loci were IGH@ (14 patients), IGL@ (14 patients), FAM46C (8 patients), IGK@ (5 patients), FOXO3 (5 patients) and BMP6 (3 patients). Several other genes of interest in B cells were identified as partners to MYC including RB1 , XBP1 , TXNDC5 , CCND3 and CCND1 . It has been suggested previously that superenhancers located at these loci upregulate their partner genes [12] , [13] . We report a significant negative correlation of MYC translocations with the t(4;14) (Bayesian inference correlation=−0.13, Bayes factor (BF)=2.11) and positive correlation with the HRD group (Bayesian inference correlation=0.13, BF=1.55). Based on these results we describe MYC translocations as being the most common translocation in myeloma and they are associated with impaired clinical outcomes ( Fig. 1a–d ). MYC translocations are an independent poor prognostic marker when analysed in multivariate analyses. Figure 1: MYC abnormalities affect survival. Progression free ( a ) and overall survival ( b ) of patients with MYC translocation, gain or no abnormality. Progression free ( c ) or overall survival ( d ) of patients comparing no MYC abnormality to those with either a translocation or gain of the locus. ( e ) relative expression of MYC in samples with no MYC abnormality, a translocation at 8q24 or gain or loss of the MYC locus. The box and whisker plot shows the 10 and 90 percentiles (whiskers) and the median and 25 and 75 percentiles (box). P values determined by log-rank test. Full size image We used CN data, generated from multiplex ligation-dependent probe amplification, to identify additional abnormalities at the MYC locus. There was a translocation involving the MYC locus in 18.4% of patients. There was a gain in 81 patients (19%), which can be subdivided into those also with a translocation (31 patients) and those with focal or chromosomal gain alone (50 patients). Combined, there was a MYC translocation or gain in 135 (32%) patients. Amplification of MYC (more than four copies) was not detected in this data set. We examined the expression of MYC in these samples and found a significant increase in expression in samples with a MYC translocation compared with those with no abnormality ( Fig. 1e ). Gains and deletions were not associated with significant increases in expression of MYC . There was no difference in the expression of MYC between samples where the translocation partner was an Ig locus and those which were non-Ig loci ( Supplementary Fig. 2 ), but there was a significant difference in OS between those with an Ig locus partner and those with a non-Ig locus partner (log rank P =0.04, Supplementary Fig. 2 ). If MYC translocated samples are removed from the data set, expression of MYC alone is not sufficient to result in a significant difference in progression free (PFS) and overall survival (OS). Kataegis co-localizes with MYC translocation breakpoints We were also able to detect a mutational signature, kataegis, where regional clustering of mutations can be indicative of somatic genomic rearrangements [14] . It is difficult to detect kataegis using exome sequencing but the tiled regions surrounding the IGH , IGK , IGL and MYC loci could be used to detect it. By creating rainfall plots, we were able to discern samples with regional hypermutation. As expected, the Ig loci contained clusters of hypermutation, but these were not enriched for C>T or C>G mutations within a TpCpH trinucleotide context and as such are not caused by kataegis. We found the hallmarks of kataegis in 15 samples (3.2%), where there was enrichment for TpCpH mutations with an inter-mutational distance <1 kb ( Fig. 2 ). Of these 15, 9 were found in the tiled region surrounding MYC and others were detected on chromosomes 1, 10, 11, 16 and 17. Kataegis was co-localized with CN abnormalities in 12 of the samples. Two of the samples with kataegis surrounding MYC also had an inter-chromosomal translocation at MYC involving either IGK or IGL . Interestingly, the partner chromosomes also showed signs of kataegis, for example, in the t(2;8) kataegis was found at IGK and MYC and in the t(8;22) kataegis was found at MYC and IGL ( Fig. 2 ). The pattern of mutations clustered around the translocation breakpoint and according to the cancer cell fraction (CCF) were present in all cells, indicating that kataegis most likely occurs at the same time as the translocation. APOBECs are thought to be involved in the generation of kataegis and as such this co-localization is indicative of APOBEC involvement in the generation of MYC breakpoints. 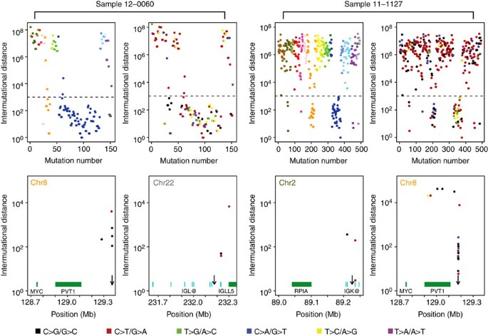Figure 2: Kataegis in myeloma. Kataegis at 8q24 coincides with translocation breakpoints and occurs on both chromosomes where a translocation has occurred. Examples of two samples are shown. For each sample the top left plot shows the distances between mutations and are coloured on a chromosomal basis according to UCSC colouring. The top right panel show the same data but is coloured by mutation type, as per the key. The bottom panels show the location on chromosome 8 and the partner translocation chromosome (22 or 2, respectively), where kataegis is found with genes or Ig loci segments indicated in green or cyan, respectively. The arrows indicated the position of the translocation breakpoint. Figure 2: Kataegis in myeloma. Kataegis at 8q24 coincides with translocation breakpoints and occurs on both chromosomes where a translocation has occurred. Examples of two samples are shown. For each sample the top left plot shows the distances between mutations and are coloured on a chromosomal basis according to UCSC colouring. The top right panel show the same data but is coloured by mutation type, as per the key. The bottom panels show the location on chromosome 8 and the partner translocation chromosome (22 or 2, respectively), where kataegis is found with genes or Ig loci segments indicated in green or cyan, respectively. The arrows indicated the position of the translocation breakpoint. 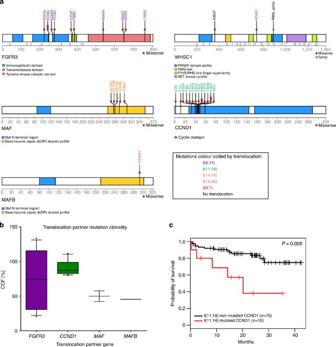Figure 3: Mutations in translocation partner oncogenes. (a) Non-synonymous mutations in translocation partner oncogenes are depicted along with the translocation group they occur in. (b) The cancer cell fraction (CCF) in which the mutations occur. (c) Mutation ofCCND1in t(11;14) samples results in decreased overall survival in Myeloma XI samples. The box and whisker plot show the 10 and 90 percentiles (whiskers) and the median and 25 and 75 percentiles (box). Full size image Hypermutation of translocation partner oncogenes In agreement with previous studies [15] , we find that CCND1 is mutated, and this was seen in 10 patients, all of whom have a t(11;14) ( Supplementary Table 3 ). All mutations occurred in the first exon of CCND1 and all but one were located outside of the cyclin box fold domains. Five patients had multiple mutations and the K50R mutation was detected in three samples, the K46N mutation was seen in two samples but all of the other mutations we describe were unique. There was no association of mutation in CCND1 with type of breakpoint (RAG or switch mediated) or allele of the variant associated with the t(11;14). There was a significant association with mutation of CCND1 and the distance to the translocation breakpoint, where samples with a breakpoint closer to CCND1 were more likely to have mutations within CCND1 ( P =0.03; Supplementary Fig. 3 ). There was also an association of mutated CCND1 and a poor prognosis when compared with non-mutated t(11;14) patients (OS median of 20.2 months versus not reached, log rank P =0.005; Fig. 3c ) in the Myeloma XI trial. This effect was also seen when comparing patients with mutated CCND1 to all other patients in the cohort and was an independent prognostic factor for both PFS and OS. To determine the significance of this result, we sequenced the first exon of CCND1 in 102 t(11;14) samples from the Myeloma IX trial and found mutations in a further 10 samples (9.8%; Supplementary Fig. 4 ). There was no effect on survival in the Myeloma IX data set with mutations in CCND1 . We also examined the allelic frequency of the variant associated with the t(11;14), rs9344, in the Myeloma XI data set and found that in agreement with our previous observations [8] the G allele is significantly associated with the translocation ( Supplementary Table 2 ). Figure 3: Mutations in translocation partner oncogenes. ( a ) Non-synonymous mutations in translocation partner oncogenes are depicted along with the translocation group they occur in. ( b ) The cancer cell fraction (CCF) in which the mutations occur. ( c ) Mutation of CCND1 in t(11;14) samples results in decreased overall survival in Myeloma XI samples. The box and whisker plot show the 10 and 90 percentiles (whiskers) and the median and 25 and 75 percentiles (box). Full size image Given the association of mutated CCND1 in the t(11;14) we examined the other translocation groups and their associated partner chromosome oncogenes. We found that FGFR3 , MAF and MAFB all had mutations which were restricted to the relevant translocation group (16.9% mutated FGFR3 in t(4;14); 12.5% mutated MAF in t(14;16) and 25% mutated MAFB in t(14;20); Fig. 3a ). There were no mutations in CCND3 (in six t(6;14) patients) and the mutations in MMSET were not in t(4;14) patients. In contrast to the poor prognosis associated with mutations of CCND1 in the t(11;14), no poor prognosis was associated with mutations in FGFR3 , MAF or MAFB . However, the latter two sample sets may be too small to address this question adequately. The mutated oncogenes were all on the der(14) and most likely reflect somatic hypermutation events mediated by AID, a member of the APOBEC family, which would normally affect the V(D)J rearrangement upstream of the IGH constant regions. After the translocation event, MMSET is on the der(4) and is, therefore, unlikely to be mutated by this mechanism. To determine that AID may be responsible, we examined the transition/transversion ratio and the proximity of the mutations to the AID consensus motif, WRC. In agreement with previous studies [16] the mutations in the IGH translocation partner genes are 58.8% in A:T bases, of which 50% are transversions ( Supplementary Fig. 5 ), and in close proximity to WRC motifs ( Supplementary Table 3 ), indicating that AID is involved in this mutational process. As AID is associated with hypermutation of the V(D)J and switch regions of the highly expressed IGH locus, we examined the expression of the translocation partner oncogene between those with or without a mutation, but found no significant differences ( Supplementary Fig. 6 ). The CCF in which the mutation was found differs by translocation group ( Fig. 3b ). In the t(11;14), the mutations were founder events present in all of the cells, whereas in the t(14;16) and t(14;20) the mutations were in only ∼ 50% of the cells, indicating they are obtained later than the translocation themselves. In the t(4;14), the mutations in FGFR3 can be either clonal or subclonal, indicating that these mutations can develop at the same time as the translocation or at a later time point. The mutation patterns for each of the der(14) oncogenes differ. In the t(11;14), mutations in CCND1 occur solely near the N terminus of the protein. In MAF and MAFB , the mutations are constrained in the basic-leucine zipper domain at the C-terminal of the protein. The focussed mutation profile seen in CCND1 , MAF and MAFB are indicative of activating mutations. The mutations in FGFR3 are dispersed through several domains but have also been described as mutations that can activate the RAS/MAPK pathway in urothelial cancer and myeloma ( Supplementary Fig. 7 ) [17] , [18] . APOBEC mutations are enriched in ‘maf’ translocation groups It has previously been shown that mutations can be described in a specific trinucleotide context and that in myeloma there are two signatures that predominate [10] . We are able to recapitulate these two different signatures, which consist of a generic signature comprised of enrichment of C>T transitions in a CpG context, Signature A ( Fig. 4a ) and a second signature, Signature B, in which there is enrichment for C>G and C>T, especially in a TpCpA context. Signature B is hypothesized to result from aberrant APOBEC activity, where the APOBECs enzymatically modify single-stranded DNA. AID is a member of the APOBEC family and is involved in class-switch recombination and somatic hypermutation in B cells. 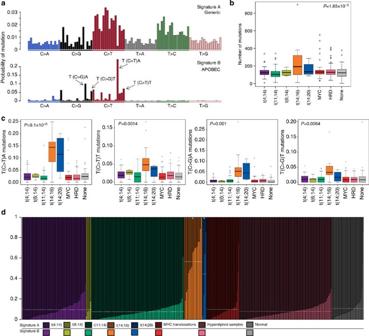Figure 4: Analysis of mutation context identifies two signatures in myeloma. (a) Mutation context identifies two signatures in myeloma, Signature A and Signature B. (b) t(14;16) and t(14;20) samples have significantly more mutations than other translocation groups. (c) The mutational context split by translocation group identifies t(14;16) and t(14;20) with more mutations which make up Signature B. (d) Stacked bar chart showing the percentage contribution of the two signatures identified by NMF in each sample, ordered by translocation group. The box and whisker plots show the 10 and 90 percentiles (whiskers) and the median and 25 and 75 percentiles (box).Pvalues determined by analysis of variance. Figure 4: Analysis of mutation context identifies two signatures in myeloma. ( a ) Mutation context identifies two signatures in myeloma, Signature A and Signature B. ( b ) t(14;16) and t(14;20) samples have significantly more mutations than other translocation groups. ( c ) The mutational context split by translocation group identifies t(14;16) and t(14;20) with more mutations which make up Signature B. ( d ) Stacked bar chart showing the percentage contribution of the two signatures identified by NMF in each sample, ordered by translocation group. The box and whisker plots show the 10 and 90 percentiles (whiskers) and the median and 25 and 75 percentiles (box). P values determined by analysis of variance. Full size image We noted that the t(14;16) and t(14;20) have a statistically significant higher number of mutations per sample compared with the other translocation subgroups (two-sided t -test P =1.65 × 10 −5 ), Fig. 4b , and that the Signature B (APOBEC) related context of mutations in the t(14;16) and t(14;20) was significantly higher than other translocation groups (T(C>T)A, P =9.1 × 10 −6 ; T(C>T)T, P =0.0014; T(C>G)A, P =0.001; T(C>G)T, P =0.0064), Fig. 4c . Collectively, mutations in these trinucleotide contexts comprise a mean of 28.7% and 21.3% of mutations in t(14;16) and t(14;20) samples, respectively (compared with t(4;14) 6.5%, t(6;14) 6.2%, t(11;14) 5.8%). We examined the proportion of each Signature present in the translocation subgroups and found that there is a significant enrichment for Signature B (APOBEC) mutations in the t(14;16) and t(14;20) (0.56, P =2 × 10 −16 ; 0.44, P =8.26 × 10 −11 , respectively) compared with the t(4;14), t(6;14), t(11;14) and HRD samples (0.094, 0.096, 0.074, 0.098 and 0.078, respectively) ( Fig. 4d ). These data indicate that the ‘maf’ translocation groups are largely characterized by APOBEC signature mutations and have a higher mutation load than the other translocation groups. To determine if there are some samples in the other translocation groups which also have an APOBEC signature, we assigned each sample to either Signature A or Signature B depending on the proportion of mutation type in each sample. This generated clusters of samples whose mutations are either mostly Signature A (cluster A) or Signature B (cluster B), Fig. 5a . Here we find that the t(14;16) and t(14;20) cases comprise 66.6% of cluster B but only 1.3% of cluster A. In line with the proportion of ‘maf’ samples in Cluster B the number of mutations in this cluster is significantly higher than in Cluster A (mean 295.44 versus 127.22, two-sided t -test, P =1.18 × 10 −15 ; Fig. 5b ). Cluster A is comprised of 445 patients and cluster B 18 patients, indicating that Signature B only affects 3.9% of patients. However, when we performed survival analysis of these patient clusters we find that there is a significant effect on OS (log rank P =0.02; Fig. 5c ). Due to the low number of samples with ‘maf’ translocations and the interaction of the translocation, APOBEC signature and mutational load this effect on survival is not significant in a multivariate analysis as it is not possible to delineate whether this effect on survival is due to any single one of these markers alone and it remains more likely that the impact of three abnormalities is linked. 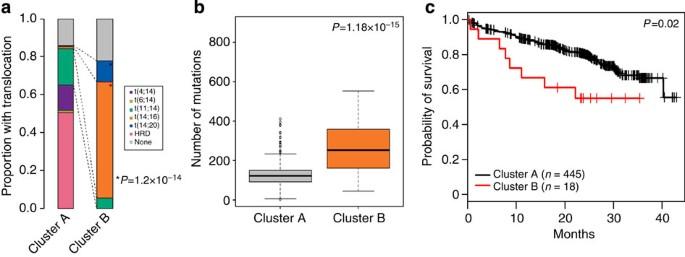Figure 5: Myeloma mutations can be categorized as belonging to Signature A or Signature B. (a) Samples which mostly have Signature B mutations dominate Cluster B and are enriched for t(14;16) and t(14;20).Pvalue determined by a linear model. (b) Samples in Cluster B have more mutations than those in Cluster A,Pvalue determined by analysis of variance. Patients in Cluster B have a significantly worse overall survival,Pvalue by log-rank test (c). The box and whisker plot shows the 10 and 90 percentiles (whiskers) and the median and 25 and 75 percentiles (box). Figure 5: Myeloma mutations can be categorized as belonging to Signature A or Signature B. ( a ) Samples which mostly have Signature B mutations dominate Cluster B and are enriched for t(14;16) and t(14;20). P value determined by a linear model. ( b ) Samples in Cluster B have more mutations than those in Cluster A, P value determined by analysis of variance. Patients in Cluster B have a significantly worse overall survival, P value by log-rank test ( c ). The box and whisker plot shows the 10 and 90 percentiles (whiskers) and the median and 25 and 75 percentiles (box). Full size image Knockdown of MAF and MAFB decreases APOBEC expression Both the t(14;16) and t(14;20) result in overexpression of a maf transcription factor. As these translocation groups are enriched for APOBEC signature mutations, we sought to determine if there is a link between maf gene expression and APOBEC expression. We examined two well-characterized gene expression data sets from myeloma patients (UAMS, GSE4581; MRC Myeloma IX, GSE15695) for characteristic expression patterns of APOBEC genes in t(14;16) and t(14;20) groups. We found that there is significantly increased expression of APOBEC3A and APOBEC3B in t(14;16) and t(14;20) cases in both the UAMS and Myeloma IX data sets ( Fig. 6 ). 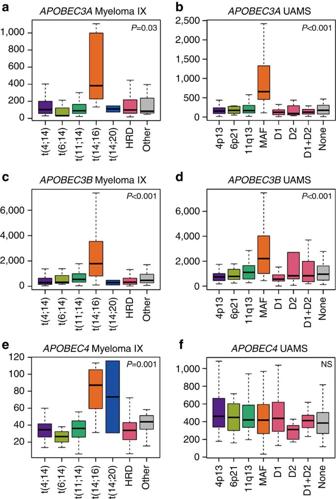Figure 6: t(14;16)/MAF samples have increased expression of APOBEC genes in the Myeloma IX (GSE15695) and the UAMS data sets (GES4581). APOBEC3A(210873_x_at) andAPOBEC3B(206632_s_at) were tested for increased expression in the t(14;16)/MAF samples and the significant results shown.Pvalue by analysis of variance. Figure 6: t(14;16)/MAF samples have increased expression of APOBEC genes in the Myeloma IX (GSE15695) and the UAMS data sets (GES4581). APOBEC3A (210873_x_at) and APOBEC3B (206632_s_at) were tested for increased expression in the t(14;16)/MAF samples and the significant results shown. P value by analysis of variance. Full size image To investigate the possibility that maf expression controls APOBEC expression, we knocked down either MAF or MAFB in RPMI-8226 (t(14;16)) or Sachi (t(14;20)) cell lines, respectively. Quantitative gene expression analysis of the cell lines indicated that only APOBEC3B was expressed in RPMI-8226 and only APOBEC4 was expressed in Sachi. In the knockdowns, we show that decreased expression of MAF results in decreased APOBEC3B expression and knockdown of MAFB results in decreased expression of APOBEC4 ( Fig. 7 ), indicating a causative link between the two sets of genes. 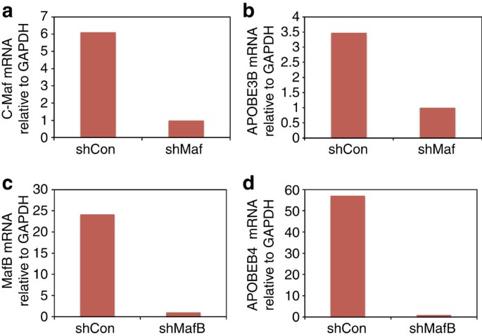Figure 7: Knockdown of MAF and MAFB by short hairpin RNAs (shRNAs) induced decrease in the expression of APOBECs. RPMI-8226 cells (a,b) were transiently infected with supernatant containing control shRNA (shCont) or shRNA specific for c-Maf (shMaf) for 48 h. Total RNA was then isolated and subjected to qRT–PCR analysis to detectMAFmRNA (a) andAPOBEC3BmRNA (b). Sachi cells (c,b) were transiently infected with supernatant containing control shRNA (shCont) or shRNA specific forMAFB(shMafB) for 48 h and expression ofMAFB(c) andAPOBEC4(d) were analysed. Figure 7: Knockdown of MAF and MAFB by short hairpin RNAs (shRNAs) induced decrease in the expression of APOBECs. RPMI-8226 cells ( a , b ) were transiently infected with supernatant containing control shRNA (shCont) or shRNA specific for c-Maf (shMaf) for 48 h. Total RNA was then isolated and subjected to qRT–PCR analysis to detect MAF mRNA ( a ) and APOBEC3B mRNA ( b ). Sachi cells ( c , b ) were transiently infected with supernatant containing control shRNA (shCont) or shRNA specific for MAFB (shMafB) for 48 h and expression of MAFB ( c ) and APOBEC4 ( d ) were analysed. Full size image Analysis of ENCODE data indicates a MAFK binding site in the promoter of APOBEC3A and APOBEC3B . Although MAFK is a different class of maf transcription factor it shares a binding motif with MAF and MAFB, which could explain the overexpression of APOBECs in the t(14;16) samples. Previously, APOBEC3B has been associated with C>T transitions in breast cancer, [19] , [20] and given that APOBEC3B is significantly overexpressed in t(14;16) or MAF group samples in both data sets this is the most likely causative candidate for the C>T transitions observed in our Signature B cases. Translocations involving the Ig loci in myeloma are recognized as primary events, being present in all cells, whereas CN abnormalities and somatic mutations tend to be present in sub-clones [21] , [22] . Here we identify translocations involving MYC as being the most common structural chromosomal abnormalities in myeloma, bringing the total translocated group to 50.1% of presenting patients and in addition MYC translocations are associated with adverse clinical outcomes. Furthermore, we show that when CN abnormalities are taken into account, the percentage of myeloma cases where MYC is deregulated is 55%, making it the most common genetic event in myeloma, being even more common than mutational activation of the RAS pathway. This observation on presenting clinical cases is consistent with previous work using myeloma cell lines and patients, which suggested that MYC deregulation is more or less ubiquitous and is mediated by non-physiological DNA damage and repair pathways [13] . In contrast, we show that in clinical samples the MYC translocation partner is an Ig locus in 30% of cases and in the remainder it is mediated by translocations to genes expressed at this stage of B-cell differentiation. While we were able to demonstrate frequent CN change at the MYC locus, using exome sequencing we were unable to gain additional mechanistic information as to why these events were occurring. From both a clinical and aetiological standpoint the positive association of MYC translocations with HRD is important because it not only reduces the size of the group where HRD is the primary aetiological factor but it also removes poor prognostic cases from this group. Tiling of the MYC and IG loci enabled us to identify a second mutational signature, kataegis, when translocations occurred between the two loci. This signature is distinct from the APOBEC signature and results in closely spaced mutations often surrounding DNA damage breakpoints. We identified two samples with the kataegis signature, which also had MYC translocations and in these cases the kataegis signature was present on both partner chromosomes, indicating that the mutational signature and the translocation co-occurred. The mechanism resulting in kataegis is not known but may also be related to the APOBECs [14] . The presence of kataegis in the MYC region is of interest because it suggests a relationship between it and the development of translocations and CN abnormalities at this site. As initiating events, translocations are poised to control the fate of the cell and ultimately of the patient, and as such it is not surprising to find that they drive the mutational pathogenesis of the disease. We find that the translocation partner oncogene is mutated in 11–25% of samples, depending on the translocation. We show that MMSET is not mutated following translocation in the t(4;14), presumably because the site of the breakpoint results in this gene being carried on the der(4) chromosome and not the der(14) as is the case with FGFR3 , CCND1 , MAF and MAFB . There is evidence to show that the mutations on the partner oncogenes are mediated by AID (distance to WRC motif and A:T mutation rate) and so they are most likely mediated via aberrant somatic hypermutation as a consequence of AID, which would normally mutate the functional V(D)J rearrangement on chromosome 14. AID is a member of the APOBEC family that deaminates C to U in actively transcribed immunoglobulin variable and switch regions resulting in somatic hypermutation through recruitment of error prone polymerases that mutate the surrounding bases through mismatch repair and base excision repair. It is not clear why only a proportion of the translocation partner genes are mutated. However, a similar situation is seen in mantle cell lymphoma, which also harbours a t(11;14). In this B-cell malignancy, mutation of CCND1 is also detected in a subset (35%) of cases and is associated with SOX11-negative and IGHV -mutated mantle cell lymphoma, suggesting their acquisition in the germinal centre [23] . These mutations are also restricted to the first exon of CCND1 , consistent with them developing as a consequence of a similar mechanism as that seen in myeloma. Interestingly, in terms of the timing of development, the mutations are clonal in t(11;14) and in some t(4;14) myeloma samples, but are subclonal in t(14;16) and t(14;20), indicating that they were acquired subsequent to the translocation. As the mutations in the partner oncogenes are mediated by AID, it raises the question as to whether they are simple passenger variants or whether they are driver events providing a selection advantage. Importantly the mutations are not randomly distributed within the partner oncogenes. In CCND1 , they are restricted to the 5′ end of the gene, outside the cyclin domain. In MAF and MAFB , the mutations are only seen in the basic-leucine zipper domain, whereas in FGFR3 they are scattered throughout the gene. Interestingly in terms of their pathological relevance, although the mutations in FGFR3 look random there is evidence that these are involved in activation of FGFR3 and downstream signalling of the RAS/MAPK pathway [18] . Many of the mutations in FGFR3 result in acquisition of a cysteine residue, often involved in di-sulphide bond formation, which may result in homo-dimerization and activation of the molecule [24] . Mutations in FGFR3 also included the K650 mutation, which constitutively activates the receptor [25] . Importantly, several of these mutations (Y373C and K650E) are present in myeloma cell lines and have been shown to result in constitutive activation of the RAS/MAPK pathway [17] . We conclude, therefore, that these mutations have been positively selected for their importance in the pathogenesis of the disease and could be targeted therapeutically. The major difference between the CCND1 and FGFR3 mutations is the effect on patient survival. However, this may not be surprising as FGFR3 activates the RAS/MAPK pathway and no effect on survival has been shown with RAS/MAPK pathway mutations ( NRAS , KRAS and BRAF ) with current treatments even though they are present in ∼ 50% of patients. Mutations in cancer samples can be subdivided based on the context of the surrounding bases. Two signatures have previously been identified in myeloma, the second of which is an APOBEC signature, and here we have been able to identify a specific genomic subgroup affected by this signature. APOBECs are a family of DNA editing enzymes, which mostly act on single-stranded DNA through deamination of cytosine to uracil [26] . As such, they have a characteristic pattern of mutation, which results in enrichment from C>G and C>T mutations in a TpCpH context. Here we find this signature in 18 of the 463 samples and these samples are highly enriched for the maf translocations, t(14;16) and t(14;20). These samples in turn also have a higher mutation load than the other samples and the samples with this signature have an adverse PFS and OS. While the t(14;16) and t(14;20) have been shown to be adverse prognostic previously [27] , [28] , [29] , the mechanism by which this is mediated has been unclear. It is known that the t(14;16) and t(14;20), as well as the t(4;14) result in the indirect upregulation of CCND2 3 but the relationship of this to adverse outcomes is undetermined. Here, we show that the t(14;16) and the t(14;20) have more mutations than other cytogenetic groups of myeloma, these mutations have an APOBEC signature, and they overexpress APOBEC genes, specifically APOBEC3A and APOBEC3B . The common mechanism between the two different translocation groups is that they result in overexpression of a maf transcription factor ( MAF or MAFB ). Interestingly, examination of ENCODE data shows maf binding sites in the promoter regions of APOBEC3A and APOBEC3B , giving a link between the translocations and the increase in mutation load and type. APOBEC3B has also been implicated in the APOBEC mutational signature in breast, ovarian and multiple other human cancers, consistent with these data [19] , [20] , [30] . It is interesting to note that the presence of t(14;16) or t(14;20) in pre-malignant MGUS and asymptomatic myeloma is associated with a favourable prognosis and a long time to progression to myeloma in contrast to when they are seen in myeloma [9] . Given the high mutational burden of this subgroup it will be important to determine if the mutational signature seen in the maf subgroups is also present at the MGUS stage, or whether the signature only manifests when the disease has progressed to myeloma. Here we show three different mutational signatures mediated by the APOBEC family: translocation partner mutation by AID, Signature B (APOBEC) mediated by APOBEC3A or APOBEC3B and kataegis mediated by an unknown APOBEC family member. We also show for the first time a clinical impact of APOBEC mutations and their association with a poor prognosis. The poor prognosis of this mutational signature is inextricably linked to a high mutation load and the adverse t(14;16) and t(14;20) translocation subgroups, making it not currently possible to disentangle the individual impact of these markers on prognosis. Patient samples Samples were taken, following informed consent, from patients newly diagnosed with symptomatic myeloma and enrolled in the Myeloma XI trial (NCT01554852). The study was approved by the NHS Health Research Authority, National Research Ethics Service Committee and by local review committees at all participating centres. Experimental procedures were approved by the NHS Health Research Authority National Research Ethics Service Committee London-Surrey Borders (CCR3019). This was a large, phase III, open label trial where patients, with no age limit were randomised between triplet immunomodulatory drug induction of either cyclophosphamide, thalidomide, dexamethasone (CTD) or cyclophosphamide, lenalidomide, dexamethasone (CRD). Patients with a suboptimal response (<very good partial response) were randomised to pre-transplant treatment with a proteasome inhibitor triplet (cyclophosphamide, bortezomib, dexamethasone and CVD). Older or less fit patients had appropriate dose reductions to therapy and did not receive an autologous stem cell transplant (ASCT). All patients subsequently underwent a maintenance randomization to either no maintenance, lenalidomide maintenance or lenalidomide and vorinostat maintenance. Exclusion criteria include renal failure requiring dialysis and solitary plasmocytoma as well as the standard criterion. PFS and OS was measured from initial randomization and the median follow-up for this analysis was 25 months (95% 24.3–26.2). The patient demographics are presented in Table 1 and a diagram of the different study arms in Supplementary Fig. 8 . The median PFS was 26.6 months (95% confidence interval (CI) 23.6–29.9) and OS was not reached but the 3 years survival rate was 66% (95% CI 60%–73). Table 1 Patient demographics. Full size table CD138+ cells were isolated from the bone marrow of patients using CD138+ MACSorting (Miltenyi Biotech, Bisley, UK) to a purity >95%. Cells were lysed in RLT+ buffer and DNA and RNA extracted using the AllPrep kit (Qiagen, Manchester, UK). Peripheral blood was also isolated from patients, white blood cells purified by Ficoll-Pacque and DNA extracted from the cell pellet using the QIAamp DNA mini kit (Qiagen). RNA and DNA were quantified using the 2200 Tapestation (Agilent Technologies, Santa Clara, CA) and Pico-green (Life Technologies, Paisley, UK). Multiplex ligation-dependent amplification About 50 ng of sample DNA was subjected to MLPA reactions using the SALSA P425-B1 probemix developed by MRC-Holland (Amsterdam, The Netherlands) [31] . The probemix contained 46 probes for CN analysis of the major prognostic markers in myeloma including: 1p32-31 ( FAF1, CDKN2C, PPAP2B and DAB1 ), 1p21, 1p12 ( FAM46C ), 1q21.3 ( CKS1B ), 1q23.3, 5q31.3, 12p13.31 ( CD27, CHD4 ), 13q14 ( RB1, DLEU1, DLEU2, DIS3 ), 16q12 ( CYLD ), 16q23 ( WWOX ) and 17p13 ( TP53 ). In addition, 11 reference probes were also included, analysing various autosomal chromosome loci, which are only infrequently involved in CNA in myeloma. A second panel was used to interrogate the MYC locus, which contained probes for exons 1 and 3. The MLPA reaction, including internal quality controls and negative controls, was performed according to manufacturer’s instructions. The PCR products were analysed using an ABI 3730 DNA analyzer (Life Technologies) and Coffalyser software (MRC-Holland, Netherlands). After intra-sample and inter-sample normalizations, CN at each locus was estimated [32] . In summary, values ≥1.2; between 1.19 and 0.71; and ≤0.7 were considered as gain, normal and deletion, respectively. If multiple probes per gene were examined, a consistent result between them was required (two probes with the same result or majority of probes with same result depending on the locus/chromosome examined) [33] . Gene expression Translocations were defined using the translocation/cyclin classification based on expression of the Ig-partner oncogene. In addition, MYC expression was assayed (Hs00153408; Life Technologies) using quantitative real-time PCR (qRT–PCR) and relative quantitative values were compared with the endogenous control ( GAPDH ). Exome sequencing and analysis DNA from both tumour and peripheral blood samples were used in the exome capture protocol as previously described [34] . Briefly, 200 ng DNA was fragmented on a Covaris E-Series using the settings suggested in the Sureselect XT Target Enrichment System for Illumina Paired-End Sequencing Library protocol (version 1.5). DNA was end-repaired, A-tailed and adaptors ligated using the NEBNext DNA library prep master mix set for Illumina (New England Biolabs, Hitchin, UK). Adaptor-ligated DNA was amplified using the NEBNext High-fidelity PCR master mix (New England Biolabs) using seven PCR cycles and 750 ng DNA hybridized against RNA baits overnight (SureSelect Human All Exon V5, Agilent Technologies). The RNA baits were designed against the human exome with the addition of custom baits that tiled the IGH , IGK , IGL and MYC loci to detect the major translocations in myeloma. After hybridization, the captured DNA was indexed and amplified using Herculase II fusion DNA polymerase (Agilent Technologies) for eight PCR cycles. Four exome samples were pooled and run on one lane of a HiSeq 2000 (Illumina, Hinxton, UK) using 76-bp paired-end reads. Data quality metrics and processing FastQC (v0.10.0) was used for basic quality control of Illumina paired-end sequencing data. These files were aligned to the reference genome (GRCh37), using BWA (v.0.5.9) followed by Stampy (v.1.0.20) to improve gapped alignment. BAM files were recalibrated using GATK (v2.3.9) and deduplicated using Picard (v.1.85). Tumour and normal samples were realigned as pairs using the GATK indel realigner to improve indel call rates. Calls from a panel of 6668 highly variable SNPs within the exome capture were compared between the tumour and normal samples to confirm that they were correctly paired. Somatic mutation calling Single nucleotide variants (SNVs) were called using MuTect (v1.1.4). They were further filtered using the following criteria: minimum of 10 × depth at that site in both tumour and normal BAMs, a minimum of 1 non-reference base call in both directions, a mean Phred quality score of >26 for that base in the tumour sample, a mean mapping quality score of ≥50 across all reads at that site in the tumour sample, and the site must be uniquely alignable according to the CRG alignablity tracks available from the UCSC genome browser and created using the GEM mappability tool (Fast Computation and Applications of Genome Mappability by Derrien et al , 2012) [35] . C>A|G>T SNVs likely to be oxidation artefacts created during library preparation were removed [36] . Short indels were called using the GATK Indelocator and furthered filtered according to the following criteria: a minimum of 1 non-reference base call in both directions, a mean Phred quality score of >26 for that base in the tumour sample, a mean mapping quality score of ≥50 across all reads at that site in the tumour sample, and the site must be uniquely alignable. No more than two reads covering that site in the normal sample could contain any indel. A window of 21 bp centred on the first base of the indel was taken and had to conform to the following rules, which remove low complexity sequences: no homopolymers of >6 bp and no dinucleotide may occur more than five times. Deletions of whole exons (windows defined as the regions used in the Agilent exome capture) were found by comparing the read depth between the tumour and normal samples. The mean depth across the window was required to be >0.2 of the median depth in the normal sample and <0.06 in the tumour sample, with the normal value being at least 8 × greater than the tumour value. CN across the exome was determined using Control-FREEC [37] utilizing 500 bp bins, each overlapping with the subsequent and previous 250 bp. A minimum average read depth of 50 was required in the control samples, with at least two neighbouring bins required to show CN aberration to call a region as gained or lost. All somatic events were annotated using both SnpEff (v3.1) and Oncotator (v0.4.2.2) with SnpEff providing the most deleterious interpretation regardless of transcript and Oncotator annotating only the canonical transcript. Significantly mutated genes were detected by providing all SNV and short indels to the MutSigCV (v1.4) algorithm. A q -value cutoff of 0.1 was used. The proportion of tumour cells containing an SNV was calculated using the following equation: CCF =cancer cell fraction (proportion of cells containing the mutation) CN =copy number at that site r =number of reads containing the mutation at that site R =total number of reads at that site Translocations were called using Delly [38] and manually curated in the Integrative Genomics Viewer (IGV). Translocations were considered real when there were at least 10 supporting reads and if no translocations were also found in the peripheral blood sample. Simultaneously, translocations were determined by qRT–PCR using defined cutoffs for expression of each partner oncogene [39] . Results from both techniques were compared and a consensus translocation call was generated. There was concordance between assays in 93.4% of cases. When assays were not concordant the data were examined and a decision was made. Nonnegative matrix factorization Nonnegative matrix factorization (NMF) using the NMF package in R was used to factorize a matrix of frequency of trinucleotide mutation contexts per sample, to identify underlying mutation signatures among all mutations in the 463 samples [10] , [14] . The algorithm was run between 2 and 18 underlying signatures, with 10 runs at each number. Two signatures were selected as the optimum number of signatures based around a number of quality control metrics. Samples were clustered using the consensus hierarchical clustering procedure implemented in the NMF package. Correlation studies To determine correlation between cytogenetic abnormalities a probabilistic approach based on Bayesian interference was determined in R [40] using the programme ‘JAGS’ [41] and it is the R interface Bayesmed [42] as previously described [43] . The probability of the observed data under the null hypothesis versus the alternative hypothesis or BF was computed. BF>1 was considered significant. Survival analysis Survival analysis was performed in R 39 using package survival [44] , [45] and coin [46] , [47] Differences between curves were tested for statistical significance using the log-rank test, with P <0.05 taken as the level of significance. Cell lines and cell culture Sachi is a cell line derived from a t(14;20) primary plasma cell leukaemia with increased levels of MAFB transcripts and was derived by Hanamura et al [48] , [49] . RPMI-8226 is a cell line obtained from the ATCC with a t(14;16) translocation and increase levels of MAF transcripts [50] . RPMI-8226 and Sachi were cultured in RPMI1640 (Invitrogen, Carlsbad, CA) containing 10% heat-inactivated foetal bovine serum and 4 mM L-glutamine, as described previously [51] . 293T cells were cultured in Dulbecco Modified Eagle Medium containing 10% heat-inactivated foetal bovine serum, penicillin (100 U ml −1 ), streptomycin (100 mg ml −1 ), 4 mM L-glutamine and 1 mM sodium pyruvate. The cells were maintained at 37 °C and humidified with 95% air and 5% CO 2 for cell culture. Silencing c-maf and mafB expression by short hairpin RNA The knockdown of c-Maf and MafB genes were performed in myeloma cells [52] . Briefly, the sequence for short hairpin RNA specific to human c-MAF gene (5′-CCGGTGGAAGACTACTACTGGATGACTCGAGTCATCCAGTAGTAGTCTTCCATTTTT-3′) and to MafB (5′-CCGGGCCTTGTCTTATGGTCAAATTCTCGAGAATTTGACCATAAGACAAGGCTTTTT-3′) in lentiviral vector were transfected into 293T cells and supernatant from culture media were harvested and concentrated. A control oligonucleotide sequence not matching any sequence in the human genome (5′-GATCCCCGACACGCGACTTGTACCACTTCAAGAGAGTGGTACAAGTCGGTCGTCTTTTTA-3′) was used as a control short hairpin RNA sequence (designated as shCont). The myeloma cells were infected with lentivirus supernatants for 48 h and total RNA was isolated using TRIzol (Life Technologies) according to the manufacturer’s instructions. Real-time quantitative PCR The gene expression was detected by qRT–PCR analysis. Briefly, 1 μg of total RNA was reverse transcribed into complementary DNA (cDNA). QPCR was performed using an ABI Prism 7600 sequence detection system (Applied Biosystems, Foster City, CA). The primers specific for human c-Maf (Hs04185012_s1), MafB (forward primer 5′-gcccgaccgaacagaagac-3′, reverse primer 5′-ctcgggcgtcaggttgag-3′, probe 5′-FAM-agcagatgaacccc-MGB-3′), Apobec3a (Hs02572821_s1),-3b (Hs00358981_m1) and -4 (Hs01941751_s1) were purchased from Applied Biosystems (Paisley, UK). A reaction mixture contained 400 ng cDNA, dedicated buffers with specific primers and probes (5′-labelled by 6-carboxy-fluorescein and 3′-labelled by 1-carboxy-teteramethyrhdamine) and DNA polymerase in a total 20 μl volume. Following 2 min incubation at 50 °C and 10 min incubation at 95 °C for denaturing, the reaction was subjected to 40-cycle amplification at 95 °C for 15 s to denature and at 60 °C for 1 min for annealing/extension. Each cDNA sample was analysed in triplicate in parallel with GAPDH as a control. Changes in messenger RNA concentration were determined by subtracting the CT of target gene from the CT of GAPDH (Δ=CT gene-CT GAPDH). The mean of Δ control was subtracted from the Δtarget gene reaction (mean Δ control−Δtarget gene= e ). The difference was calculated as 2 e by the 2−ΔΔCT . Accession codes : Genome data have been deposited at the European Genome-phenome Archive (EGA, http://www.ebi.ac.uk/ega/ ) which is hosted at the EBI, under accession number EGAS00001001147. How to cite this article : Walker, B. A. et al . APOBEC family mutational signatures are associated with poor prognosis translocations in multiple myeloma. Nat. Commun . 6:6997 doi: 10.1038/ncomms7997 (2015).